Unexpectedly high pressure for molecular dissociation in liquid hydrogen by electronic simulation The study of the high pressure phase diagram of hydrogen has continued with renewed effort for about one century as it remains a fundamental challenge for experimental and theoretical techniques. Here we employ an efficient molecular dynamics based on the quantum Monte Carlo method, which can describe accurately the electronic correlation and treat a large number of hydrogen atoms, allowing a realistic and reliable prediction of thermodynamic properties. We find that the molecular liquid phase is unexpectedly stable, and the transition towards a fully atomic liquid phase occurs at much higher pressure than previously believed. The old standing problem of low-temperature atomization is, therefore, still far from experimental reach. Hydrogen is the simplest element in nature and nevertheless its phase diagram at high pressures ( P s) remains a challenge both from the experimental and theoretical points of view. Moreover, the understanding of equilibrium properties of hydrogen in the high pressure regime is crucial for a satisfactory description of many astrophysical bodies [1] and for discovering new phases in condensed matter systems. At normal pressures and temperatures ( T s), the hydrogen molecule H 2 is exceptionally stable and thus the usual phases are described in terms of these molecules, that is, solid, liquid and gas molecular phases (see Fig. 1 ). 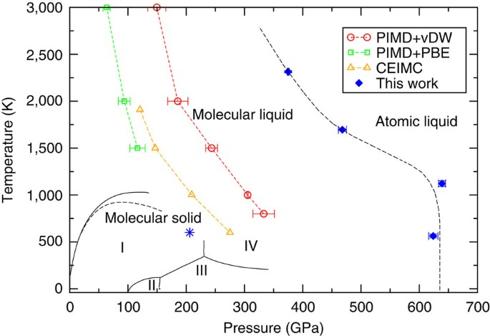Figure 1:P-Tphase diagram of hydrogen. Black solid lines indicate experimental boundaries between the molecular liquid and the molecular solid, the latter consisting of four different solid phases denoted by I, II, III and IV as in ref.11. Coloured symbols with dashed curves correspond to the liquid–liquid transition (LLT) obtained with latest simulations. Red circles and green squares refer to density functional theory (DFT) calculations with different functionals (PBE and vdW)20, while orange triangles refer to coupled electron-ion Monte Carlo (CEIMC)19,34. Blue diamonds correspond to the LLT estimated in this work. Our simulations also find that solidification occurs starting from a molecular liquid at a parameter indicated by a blue star. The black dashed line is a guide to the eye. Figure 1: P - T phase diagram of hydrogen. Black solid lines indicate experimental boundaries between the molecular liquid and the molecular solid, the latter consisting of four different solid phases denoted by I, II, III and IV as in ref. 11 . Coloured symbols with dashed curves correspond to the liquid–liquid transition (LLT) obtained with latest simulations. Red circles and green squares refer to density functional theory (DFT) calculations with different functionals (PBE and vdW) [20] , while orange triangles refer to coupled electron-ion Monte Carlo (CEIMC) [19] , [34] . Blue diamonds correspond to the LLT estimated in this work. Our simulations also find that solidification occurs starting from a molecular liquid at a parameter indicated by a blue star. The black dashed line is a guide to the eye. Full size image In the early days, it was conjectured by Wigner and Huntington [2] that, upon high pressure, this stable entity—the H 2 molecule—can be destabilized, giving rise to an electronic system composed of one electron for each localized atomic center, namely, the condition that, according to the band theory, should lead to metallic behaviour. After this conjecture, an extensive experimental and theoretical effort has been devoted, an effort that continues to be particularly active also recently [3] , [4] , [5] , [6] , [7] , [8] , where some evidence of metallicity in hydrogen has been reported. While a small resistivity has been observed in the molecular liquid state in the range of 140–180 GPa and 2,000–3,000 K (ref. 4 ), it is not clear whether this observation is above a critical temperature T *, where only a smooth metal–insulator crossover can occur, and whether metallization is due to dissociation or can occur even within the molecular phase. Evidence of a phase transition has been clearly reported in ref. 7 , though the temperature has not been measured directly. Moreover indirect evidence of a phase transition at around 120 GPa and 1,500 K has been claimed. By contrast, any indication of metallization has not been observed in the low-temperature solid phase yet [9] , [10] , [11] . Until very recently, the density functional theory (DFT) method has been considered as the standard tool for the simulation of electronic phases, because it allows the simulation of many electrons with a reasonable computational effort. However, there are several drawbacks in this technique especially for the study of the dissociation of hydrogen: (i) the single molecule is not accurately described at equilibrium and especially in the dissociation limit [12] , [13] (see Fig. 2c ). (ii) Electronic gaps are substantially underestimated [14] within DFT, implying that possible molecular phases are more easily destabilized within standard density functionals (DFs). For all the above reasons, DFT seems not adequate for the hydrogen problem under high pressure, especially in a range of pressures unaccessible by experiments, where the quality of a particular DF cannot be validated. Indeed, several DFT simulations on this particular subject [15] , [16] , [17] , [18] lead to contradictory results for the nature of the molecular liquid–atomic liquid transition, and its position in the phase diagram may vary in a range of more than 100 GPa according to different DFs [19] , [20] , [21] . Recently, it has also been shown that DFT solid stable phases strongly depend on the DF used [22] , [23] , [24] , suggesting quite clearly that the predictive power of DFT is limited for hydrogen. 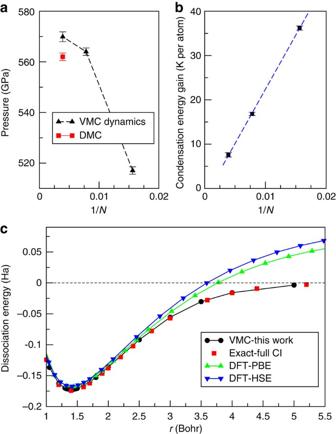Figure 2: Accuracy and finite size effects. (a) Pressure as a function of the system sizesN=64, 128 and 256 at a densityrs=1.22 (the Wigner-Seitz radiusrsis defined asV/N=4/3π(rsa0)3whereVis the volume,Nthe number of ions anda0is the Bohr radius.) near the transition at 600 K. The diffusion Monte Carlo (DMC) value, obtained from 20 equilibrated (N=256) configurations generated by the variational Monte Carlo (VMC) dynamics, is also plotted (red square). (b) Finite size scaling of the condensation energy gain atrs=1.28 and 600 K. The condensation energy gain becomes negligible in the infinite size limit (see Methods). (c) Dissociation energy curves for theH2molecule for different methods, QMC at the VMC level and with the same variational wavefunction employed in the dynamics, DFT with PBE or HSE DFs14, and the exact curve obtained with full configuration interaction (CI) method35. Figure 2: Accuracy and finite size effects. ( a ) Pressure as a function of the system sizes N =64, 128 and 256 at a density r s =1.22 (the Wigner-Seitz radius r s is defined as V/N =4/3π( r s a 0 ) 3 where V is the volume, N the number of ions and a 0 is the Bohr radius.) near the transition at 600 K. The diffusion Monte Carlo (DMC) value, obtained from 20 equilibrated ( N =256) configurations generated by the variational Monte Carlo (VMC) dynamics, is also plotted (red square). ( b ) Finite size scaling of the condensation energy gain at r s =1.28 and 600 K. The condensation energy gain becomes negligible in the infinite size limit (see Methods). ( c ) Dissociation energy curves for the H 2 molecule for different methods, QMC at the VMC level and with the same variational wavefunction employed in the dynamics, DFT with PBE or HSE DFs [14] , and the exact curve obtained with full configuration interaction (CI) method [35] . Full size image Among all first principle simulation methods, the quantum Monte Carlo (QMC) method provides a good balance between accuracy and computational cost and it appears very suitable for this problem. The QMC approach is based on a many-body wavefunction—the so called trial wavefunction—and no approximation is used in the exchange and correlation contributions within the given ansatz [25] . For instance, the exact equilibrium bond length and the dissociation energy profile for the isolated H 2 molecule are correctly recovered (see Fig. 2c ) within this approach. Only few years ago, the calculation of forces has been made possible within QMC, with affordable algorithms [26] . Therefore, very efficient sampling methods are now possible, that are based on molecular dynamics (MD), where in a single step all atomic coordinates are changed according to high-quality forces corresponding to a correlated Born-Oppenheimer energy surface (see Methods). In this way, it is possible to employ long-enough simulations that are well equilibrated and are independent of the initialization, also for very large size. With this newly developed QMC simulations, here we report numerical evidences for a first-order liquid–liquid transition (LLT) between the molecular and the atomic fluids. We find critical behaviour in pressures as a function of (isothermal) density and as a function of (isochoric) temperature. Moreover, a clear abrupt change in the radial pair distribution function at the LLT is also observed, even though molecules start to gradually dissociate well before the transition. We also find that the LLT occurs at much higher densities, hence at much higher pressures, as compared with recent calculations [19] , [20] . By looking at the steepness of the evaluated LLT boundary in the phase diagram (see Fig. 1 ), we can also give the estimate of ~600 GPa for the expected complete atomization of the zero-temperature structure. However, this remains an open issue since in our work we have neglected quantum effects on protons, which may be certainly important at low temperatures. Moreover, this quantitative prediction should hold, provided the dissociation occurs between two liquid phases down to zero temperature [27] and no solid atomic phase emerges. System size and sampling scheme We employ simulation cells containing up to 256 hydrogen atoms and use a novel MD scheme with friction in the NVT ensemble (see Supplementary Note 1 , Supplementary Fig. 1 ), for simulation times of few picoseconds, long enough to have well-converged results on the pressure, internal energy and the radial pair distribution function g ( r ). Notice also that our approximation to consider QMC in its simplest variational formulation (see Methods), that is, variational Monte Carlo (VMC), is already quite satisfactory because the much more demanding diffusion Monte Carlo (DMC) can correct the pressure only by few GPas (see Fig. 2a ), which is not relevant for the present accuracy in the phase diagram, rather size effects seem to be much more important (see Methods). In this regard, we also performed a DMC-MD on a much smaller system with 54 protons and we have verified that, apart from an overall shift in the total electronic energy, VMC and DMC dynamics give quantitatively the same results for the pressure and the g ( r ) (see Supplementary Fig. 2 , Supplementary Note 2 ). This implies that the forces, evaluated at the VMC level, are already accurate to drive the dynamics to the correct equilibrium distribution. Ergodicity of QMC simulations In our approach, we cannot address directly the issue of metallicity or insulator behaviour but can assess possible first-order transition by large-scale simulations, where any discontinuity of correlation functions with varying temperature or pressure should be fairly evident and clear. Considering that even an insulator with a true gap should also exhibit residual-activated conductivity at finite temperatures, a metal–insulator transition at finite temperatures can be experimentally characterized only by a jump (usually by several orders of magnitude) of the conductivity. Hence, without a first-order transition, namely, without discontinuous jumps in the correlation functions upon a smooth variation of temperature or pressure, we cannot define a true metal–insulator transition at finite temperatures, otherwise it is rather a crossover. To assess that our QMC method is capable of characterizing correctly a phase transition, we carefully check for the possible lack of thermalization near the phase transition by repeating the simulations with very different starting ionic configurations at the same thermodynamic point. Moreover, the functional form of the trial wavefunction is flexible enough to correctly describe both the paired and the dissociated state (see Methods), and therefore our approach is expected to be particularly accurate even for the LLT. A complete equilibration is reached within the QMC framework since no hysteresis effects occur in all the range of temperatures studied (see Fig. 3 and Supplementary Fig. 3 ). 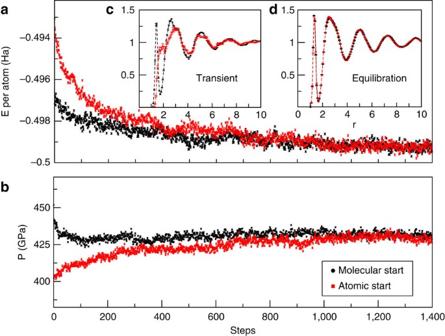Figure 3: Ergodicity of the simulations. (a) EnergyEand (b) pressurePas a function of the ionic steps during a Langevin dynamics simulation atrs=1.28 andT=600 K. Red squares refer to a simulation whose starting configuration is an atomic fluid, while black circles correspond to a molecular initial configuration (see insetcfor the radial pair distribution functions of these two configurations). After equilibration, energy, pressure and radial pair distribution function (insetd) converge to the same values. Figure 3: Ergodicity of the simulations. ( a ) Energy E and ( b ) pressure P as a function of the ionic steps during a Langevin dynamics simulation at r s =1.28 and T =600 K. Red squares refer to a simulation whose starting configuration is an atomic fluid, while black circles correspond to a molecular initial configuration (see inset c for the radial pair distribution functions of these two configurations). After equilibration, energy, pressure and radial pair distribution function (inset d ) converge to the same values. Full size image Characterizing the first-order transition To identify the LLT, we trace four isotherms in the range of 600–2,300 K, looking for a possible singular behaviour of the pressure and the radial pair distribution function g ( r ), in a wide range of density (see Supplementary Note 3 , Supplementary Fig . from 4 to 11 ). We indeed find a relatively small discontinuity, which appears to be clear also at the highest temperature considered (see Fig. 4a,b ). A similar first-order behaviour is also found by looking at the pressure as a function of temperature at fixed density (see Supplementary Fig. 12 ), that is, by crossing the LLT vertically, along the isochor having density r s =1.28. Notice that, close to the transition, a fully molecular phase is not stable, as a large fraction of pairs is found to be already dissociated ( Fig. 4b ). Our results are summarized in the P - T phase diagram shown in Fig. 1 . We should note here that, in our calculations, we neglect nuclear quantum effects. However, this approximation should slightly affect the location of the transition, as it was shown that the inclusion of the zero-point motion shifts the LLT towards smaller pressures only by about 40 GPa (refs 19 , 20 ). 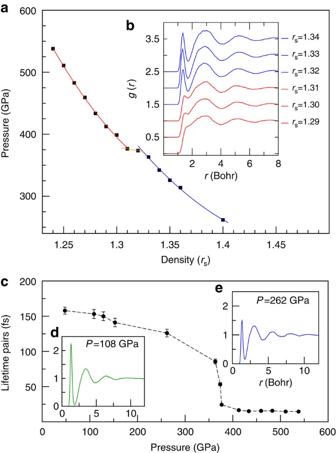Figure 4: Liquid–liquid transition at 2,300 K. (a) Pressure as a function of the density. A clear plateau is visible aroundrs=1.31−1.32, indicating the first-order transition. This evidence is also supported by the discontinuous change withrsin the radial pair distribution functiong(r) (insetb). (c) Average lifetime of pairs as a function of pressure. A pair is defined here as a couple of ions that are nearest neighbours and whose distanceris smaller than a cutoffrc=1.70 Bohr. The shape of this curve is qualitatively similar for every reasonable choice ofrc, although its amplitude may slightly vary. In the insets (d) and (e), radial pair distribution functions for two different pressures (P) in the molecular fluid. The higher the pressure, the smaller is the molecular peak and more coordination shells appear in the long-range tail. Figure 4: Liquid–liquid transition at 2,300 K. ( a ) Pressure as a function of the density. A clear plateau is visible around r s =1.31−1.32, indicating the first-order transition. This evidence is also supported by the discontinuous change with r s in the radial pair distribution function g ( r ) (inset b ). ( c ) Average lifetime of pairs as a function of pressure. A pair is defined here as a couple of ions that are nearest neighbours and whose distance r is smaller than a cutoff r c =1.70 Bohr. The shape of this curve is qualitatively similar for every reasonable choice of r c , although its amplitude may slightly vary. In the insets ( d ) and ( e ), radial pair distribution functions for two different pressures ( P ) in the molecular fluid. The higher the pressure, the smaller is the molecular peak and more coordination shells appear in the long-range tail. Full size image In the high-pressure phase diagram, our results suggest the existence of a mixed—although mainly molecular—liquid, surrounding the solid IV mixed molecular atomic phase (see Fig. 1 ). We have studied the average lifetime of the pairs formed by the nearest neighbouring hydrogen ions. As shown in Fig. 4c , it exhibits a clear jump with varying pressure at 2,300 K, supporting the location of the LLT at 375 GPa. We also notice a precursor drop of the lifetime at around 150 GPa, which corresponds to the onset of the dissociation. This value of 150 GPa is consistent with the pressure range where a drastic but continuous drop of the resistivity is observed in the molecular phase [4] . To better characterize the LLT, we study in Fig. 4d,e the dissociation fraction and the long-range behaviour of g ( r ) for two fluid configurations at pressures much smaller than the true first-order transition point. Nevertheless, a qualitative change in the behaviour of these quantities is evident even within the same phase. Remarkably, not only the dissociation fraction increases with the pressure but also the number of oscillations in the long range g ( r ) tail becomes larger, both features being very similar to what is observed in the high-pressure phase. By taking also into account that, at non-zero temperature, a finite and large conductivity can be activated, it is clear that a rather sharp variation of physical quantities can occur much before the first-order transition. In conclusion, we have reported the first description of the dissociation transition in liquid hydrogen by ab initio simulation based on the QMC method with fairly large number of atoms. The main outcomes of our study are summarized as follows: (i) the transition, which appears to be first order, occurs at substantially higher pressures than the previous ab initio predictions based on DFT. (ii) Employing QMC simulations with large number of atoms is essential because the stability of the molecular phase is otherwise underestimated. (iii) The first-order character is evident also at the highest temperatures, suggesting that even at these temperatures this transition is not a crossover. (iv) the shape of the LLT boundary is rather unusual and becomes a vertical line in the P - T phase diagram for T <1,100 K. By assuming that also at lower temperatures no solid phase emerges, the dissociation pressure should remain almost temperature independent. Therefore, even by considering an upper limit of 100 GPa shift to lower pressures, due to proton quantum effects not included here, we predict that experiments should be done at least above 500 GPa to realize the Wigner and Huntington dream of hydrogen atomic metallization. Accuracy of QMC methods In this work, we employ the QMC approach for electronic properties. In the simplest formulation, the correlation between electrons is described by the so called Jastrow factor J of the following general form where r i and r j are electron positions and u is a two-electron function to be determined variationally. It is enough to apply this factor to a single-Slater determinant to remove the energetically expensive contributions of too close electrons occupying the same atomic orbital and to obtain for instance the correct dissociation limit for the H 2 molecule (see Fig. 2c ), and essentially exact results for the benchmark hydrogen chain model [28] . Starting from this Jastrow-correlated ansatz, an important projection scheme has been developed—the diffusion Monte Carlo (DMC)—that allows an almost exact description of the correlation energy, with a full ab initio many-body approach, namely by the direct solution of the Schrödinger equation. Unfortunately, QMC is much more expensive than DFT, and so far its application has been limited to small number of atoms [19] . Variational wavefunction For the calculation of the electronic energy and forces, we use a trial correlated wavefunction of the form The determinantal part | SD › (Slater determinant) is constructed starting from N /2 molecular orbitals, N being the total number of electrons, while the Jastrow part can be written as J = J 1 J 2 J 3 . The Jastrow factor takes into account the electronic correlation between electrons and is conventionally split into a homogeneous interaction J 2 depending on the relative distance between two electrons, that is, a two-body term as in Equation 1, and a non-homogeneous contribution depending also on the electron-ion distance, included in the one-body J 1 and three-body J 3 . The exact functional form of these components is given in ref. 29 . Both the Jastrow functions and the determinant of molecular orbitals are expanded in a gaussian localized basis. The optimization of the molecular orbitals is done simultaneously with the correlated Jastrow part. We performed a systematic reduction of the basis set to minimize the total number of variational parameters. Indeed for the present accuracy for the phase diagram, a small 2 s /atom basis set is sufficient as a larger 3 s 1 p /atom basis set only improves the total energy of <1 mH per atom and leaves substantially unchanged the radial pair distribution function, that is, the atomic(molecular) nature of the fluid (see Supplementary Fig. 13 ). The value for the LLT critic pressure is not significantly affected (for the present accuracy in the phase diagram) by the choice of the basis (see Supplementary Fig. 14 ), rather the difference between QMC and DFT with PBE functional is already evident for a system of 64 atoms. We now address an issue that, in our opinion, can be extremely important in the context of hydrogen metallization. Close to a metal–insulator transition, a resonating valence bond scenario is possible and may give rise to unconventional superconductivity [30] , namely a superconductivity stabilized without the standard BCS electron–phonon mechanism. To study this interesting possibility, we have calculated the energy gain obtained by replacing the Slater determinant with a BCS type of wavefunction, both with the same form of the Jastrow factor. This quantity is known as the condensation energy [29] and is non-zero in the thermodynamic limit when the variational wavefunction represents a superconductor. Though we neglect quantum effects on protons and we have not systematically studied this issue for all densities, this VMC condensation energy (see Fig. 2b ), computed by considering about 20 different independent samples at r s =1.28 and T=600 K, is very small and decreases very quickly with N by approaching zero in the thermodynamic limit (1/ N =0). This result at least justifies the use of a simpler Slater determinant wavefunction and shows that, the quality of the wave function can be hardly improved by different, in principle more accurate, variational ansatzes. In this way, a straightforward reduction of the number of variational parameters is possible, by exploiting also the fact that matrix elements connecting localized orbitals above a threshold distance r max do not contribute significantly to the energy. Indeed, as we have systematically checked in several test cases (see Supplementary Fig. 15 and Supplementary Table 1 ), it is enough to consider r max =4 Bohr to have essentially converged results for the molecular orbitals, implying a drastic reduction in the variational space (from ≃ 40,000 parameters to ≃ 5,000 in a 256-hydrogen system). Finite size effects All the results for the LLT presented here refer to a cubic supercell at the Γ–point (see Supplementary Table 2 ) with the largest affordable number of atoms (256) to be as close as possible to the thermodynamic limit. Indeed, even though the pressure seems to converge with the size of the simulation cell, the molecular (atomic) nature of the liquid is very sensitive to the number of atoms N . This issue was previously reported in refs 21 , 31 and cannot be removed with a better k -point sampling, because this will be equivalent to enforce a fictitious periodicity to a liquid phase. In particular, the N =64 supercell simulations, even with k -point sampling, strongly favour the dissociated liquid in both DFT and QMC frameworks (see Supplementary Fig. 16 ). Thus, the critical LLT density is severely underestimated by employing supercells smaller than N =256, which is now considered a standard size in DFT simulations of liquids. The main reason of this effect is the structural frustration, requiring the use of much larger supercells, whose dimension L has to exceed the correlation length of the liquid. A possible rule of thumb consists in checking that the g ( r ) is smoothly approaching its asymptotic value 1 at r = L . Our evidences support the conclusion that a failure in dealing with the finite size effects will result in a severe underestimation of the LLT critical densities. DFT-MD simulations were performed using the QuantumEspresso code [32] . Sampling the canonical ensemble with Langevin dynamics In this study, we sample the canonical equilibrium distribution for the ions by means of a second-order generalized Langevin equation, as introduced in ref. 26 . The major advantage of this technique consists in the efficient control of the target temperature even in the presence of noisy QMC forces. Here we improve upon this scheme devising a numerical integrator that is affected by a smaller time step error (see Supplementary Note 1 ). We adopt the ground state Born-Oppenheimer approximation, namely the variational parameters, defining our wave function, are all consistently optimized at each iteration of our MD. Therefore, the electronic entropy has been neglected in all our calculations. However, we have carefully checked that this entropy contribution is clearly neglegible in the relevant temperature range studied (see Supplementary Note 4 ). As well known, hysteresis is usually found by using local updates in simple Monte Carlo schemes, which cannot be therefore reliable to determine the phase boundary of a first-order transition. Our method, based on an advanced second-order MD with friction, is instead powerful enough that very different phases can be reached during the simulation, with time scales that remain accessible for feasible computations. Indeed, we have also experienced a spontaneous solidification in a pressure and temperature range where the solid phase is expected to be stable (see Fig. 1 and Supplementary Note 5 , Supplementary Fig. 17 for details). Though this effect has been observed in a much smaller system (64 hydrogen atoms), we believe that, after the inclusion of proton quantum effects, the present method can also shed light on understanding low-temperature solid phases, which remain still highly debated and controversial in recent years [33] . How to cite this article: Mazzola, G. et al. Unexpectedly high pressure for molecular dissociation in liquid hydrogen by electronic simulation. Nat. Commun . 5:3487 doi: 10.1038/ncomms4487 (2014).